Polystyrene sulphonic acid resins with enhanced acid strength via macromolecular self-assembly within confined nanospace Tightening environmental legislation is driving the chemical industries to develop efficient solid acid catalysts to replace conventional mineral acids. Polystyrene sulphonic acid resins, as some of the most important solid acid catalysts, have been widely studied. However, the influence of the morphology on their acid strength—closely related to the catalytic activity—has seldom been reported. Herein, we demonstrate that the acid strength of polystyrene sulphonic acid resins can be adjusted through their reversible morphology transformation from aggregated to swelling state, mainly driven by the formation and breakage of hydrogen bond interactions among adjacent sulphonic acid groups within the confined nanospace of hollow silica nanospheres. The hybrid solid acid catalyst demonstrates high activity and selectivity in a series of important acid-catalysed reactions. This may offer an efficient strategy to fabricate hybrid solid acid catalysts for green chemical processes. Driven by environmental consideration and safety concerns, the replacement of hazardous and corrosive mineral acids by solid acids is one of the important tasks for green and sustainable production of chemicals [1] , [2] , [3] , [4] , [5] , [6] , [7] , [8] . Polystyrene sulphonic acid resins (PS-SO 3 H) are among the very important solid acids in industry and have been widely used in acid-catalysed reactions such as esterification, olefin hydration, etherification and alkylation of phenols [9] , [10] , [11] , [12] , [13] . They generally exhibit high concentration of acid sites but poor thermal stability and very low surface area. A straightforward strategy for improving thermal stability and for increasing surface area is to prepare polymer/silica hybrid composites, which could take advantages of high surface area, high thermal stability and antiswelling properties of silica materials via either physically mixing or covalently bonding method [14] , [15] , [16] , [17] . Although polymer/silica hybrid composites exhibit increased thermal stability, higher exposure degree of acid sites and larger BET (Brunauer-Emmett-Teller) surface area in comparison with their polymer counterparts, the acid strength of PS-SO 3 H could not be enhanced and on the contrary it might become lower because of the reduced acid density by this approach [18] . It has been reported that the increment in acid density and spatial proximity may increase the cooperative effect among acid sites, consequently enhancing the acid strength of PS-SO 3 H [19] , [20] . As for inorganic solid acids, the acid strength could be adjusted by varying several factors, for example, crystallinity, topology structure and morphology, in addition to the chemical compositions [21] , [22] , [23] , [24] , [25] , [26] , [27] . For example, microporous zeolites with crystalline nature exhibit stronger acid strength than mesoporous Al-MCM-41 with amorphous nature, even though they are both composed of aluminosilicates [21] . Recently, it has been reported that Brönsted acid strength of the titanate nanotubes is higher than that of the titanate nanosheets, which is attributed to the lattice distortion derived from scrolling of the lamellar titanate nanosheet [24] . As for the polymer-based solid acids, the principal strategy to enhance acid strength is to add electron-withdrawing groups on the sulphonated phenyl groups [27] . Great challenge still remains for improving the acid strength via factors beyond chemical compositions, probably due to the lack of methods for morphology, structure and crystalline controls of polymers. Macromolecular self-assembly that involves thermodynamically controlled association of molecules into aggregates has been widely used for the fabrication of polymers with well-defined structures [28] , [29] , [30] , [31] , [32] , [33] . Generally, the self-assembly is performed in bulk solution system via interactions among specific functional groups, for example, H-bond interactions, hydrophobic interactions, electrostatic interactions and π–π stacking. The macromolecular self-assembly in a confined nanospace has seldom been investigated and may be distinctively different from that in bulk solution system due to the confinement effect in nanospace, relatively high local concentration of substrates, restricted movement freedom of substrates and so on. Herein, we report the fabrication of a hybrid solid acid with a double-shell nanostructure (DSNs) via the self-assembly of PS-SO 3 H in the confined nanospace of silica hollow nanospheres (HNs). The acid strength of PS-SO 3 H can be reversibly enhanced and decreased by the expansion and aggregation of PS-SO 3 H within the confined nanospace, which is confirmed by 31 P MAS NMR, ammonia adsorption calorimetry and TEM (transmission electron microscopy) characterizations. In a series of important acid-catalysed reactions, such as esterification of fatty acid, Friedel–Crafts alkylation of toluene and cumene hydroperoxide (CHP) cleavage, the solid catalyst exhibits much higher activity than Amberlyst-15, and in some cases even higher than liquid acid, H 2 SO 4 , under similar reaction conditions. Morphology and nanostructure The general procedure for the synthesis of hybrid solid acid is outlined in Fig. 1a . Initially, PS template spheres with a particle size of ~200 nm were prepared by emulsion polymerization in water system ( Fig. 1b and Supplementary Fig. 1a ). Then PS@ meso silicas with yolk-shell nanostructures (YSNs) were synthesized according to a modified organosilane-assisted etching method that we reported previously using 1,2-bis-(trimethoxysilyl)ethane (BTME) as the organosilane precursor [34] , [35] . The TEM image shows that the core diameter and shell thickness of PS@ meso silicas YSNs are ~200 and ~40 nm, respectively, and the void between core and shell is ~40 nm ( Fig. 1c ). After surfactant extraction, PS@ meso silicas YSNs were sulphonated with ClSO 3 H in CH 2 Cl 2 for the formation of PS-SO 3 H@ meso silicas DSNs. The SEM image shows that PS-SO 3 H@ meso silicas DSNs are mono-dispersed nanospheres with a uniform particle size of ~340 nm, similar to YSNs before sulphonation, and the broken particles clearly show the sphere-in-sphere morphology ( Supplementary Fig. 1b ). The TEM image clearly verifies that this sample has double-shell hollow nanostructure with inner-shell thickness of ~60 nm and outer-shell thickness of ~40 nm, and the void space between the inner shell and the outer shell is of ~40 nm ( Fig. 1d ). The high-resolution-TEM element line images of PS-SO 3 H@ meso silicas DSNs clearly show that Si and S are mainly distributed in the outer shell and inner shell, respectively ( Fig. 2 ). For further identification of the composition of the outer and inner shell, PS-SO 3 H@ meso silicas DSNs were treated in HF and calcined under air atmosphere to remove silica and PS-SO 3 H, respectively. According to the TEM images, both the HF-treated and the calcined samples are HNs with the same particle sizes as the outer (~340 nm) and inner (~200 nm) HNs of PS-SO 3 H@ meso silicas DSNs ( Fig. 3a,b ). The above results demonstrate that the outer and inner shell of PS-SO 3 H@ meso silicas DSNs are composed of silica and PS-SO 3 H, respectively. 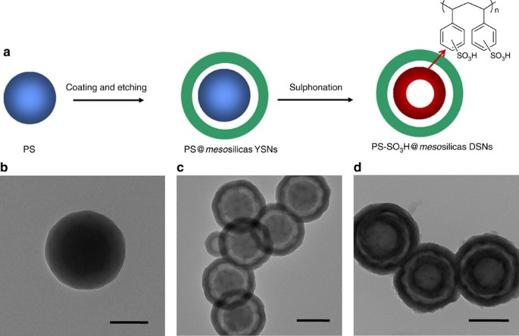Figure 1: Synthesis and characterization of PS-SO3H@mesosilicas DSNs. (a) Schematic illustration showing the general procedure for the synthesis of PS-SO3H@mesosilicas DSNs. (b) TEM image of PS template. Scale bar, 100 nm. (c) TEM image of PS@mesosilicas YSNs. Scale bar, 200 nm. (d) TEM image of PS-SO3H@mesosilicas DSNs. Scale bar, 200 nm. Figure 1: Synthesis and characterization of PS-SO 3 H@ meso silicas DSNs. ( a ) Schematic illustration showing the general procedure for the synthesis of PS-SO 3 H@ meso silicas DSNs. ( b ) TEM image of PS template. Scale bar, 100 nm. ( c ) TEM image of PS@ meso silicas YSNs. Scale bar, 200 nm. ( d ) TEM image of PS-SO 3 H@ meso silicas DSNs. Scale bar, 200 nm. 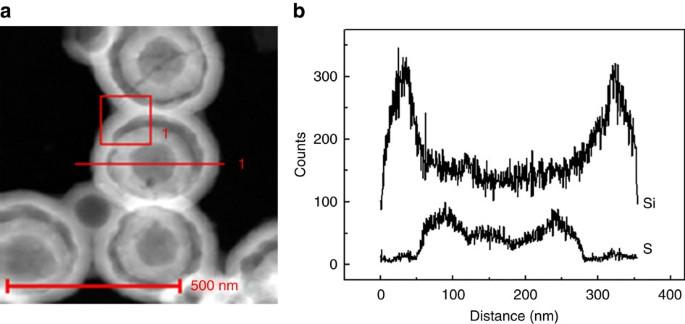Figure 2: Investigation of the PS-SO3H location. (a) High-resolution-TEM image of PS-SO3H@mesosilicas DSNs. (b) Energy dispersive X-ray spectrometer (EDX) analysis along the line shown in (a) of PS-SO3H@mesosilicas DSNs. Full size image Figure 2: Investigation of the PS-SO 3 H location. ( a ) High-resolution-TEM image of PS-SO 3 H@ meso silicas DSNs. ( b ) Energy dispersive X-ray spectrometer (EDX) analysis along the line shown in ( a ) of PS-SO 3 H@ meso silicas DSNs. 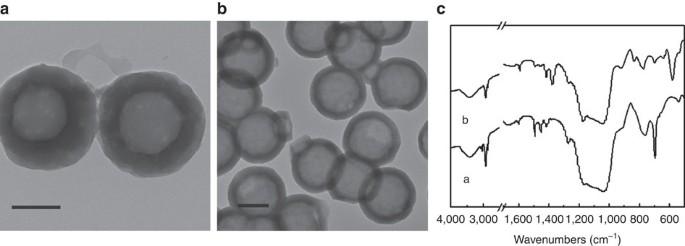Figure 3: Composition characterizations. (a) TEM image of PS-SO3H@mesosilicas DSNs after treament with HF. Scale bar, 100 nm. (b) TEM image of PS-SO3H@mesosilicas DSNs after calcinations. Scale bar, 200 nm. (c) FTIR spectra of (a) PS@mesosilicas YSNs and (b) PS-SO3H@mesosilicas DSNs. Full size image Figure 3: Composition characterizations. ( a ) TEM image of PS-SO 3 H@ meso silicas DSNs after treament with HF. Scale bar, 100 nm. ( b ) TEM image of PS-SO 3 H@ meso silicas DSNs after calcinations. Scale bar, 200 nm. ( c ) FTIR spectra of (a) PS@ meso silicas YSNs and (b) PS-SO 3 H@ meso silicas DSNs. Full size image Compositions and textural properties The appearance of the vibration peaks assigned to -CH 2 CH 2 - at 2,934–2,844 cm −1 in the FTIR (Fourier transform infrared) spectra of PS@ meso silicas YSNs and PS-SO 3 H@ meso silicas DSNs confirms the successful wrapping of the ethane-silicas around the PS cores ( Fig. 3c ). The peaks at 1,450–1,630 cm −1 and 3,000–3,100 cm −1 are assigned to unsaturated C–C and C–H stretching vibration of phenyl groups. Two new peaks at 1,178 and 1,377 cm −1 attributed to sulphonic acid groups were observed in the FTIR spectrum of PS-SO 3 H@ meso silicas DSNs. Compared with that of PS@ meso silicas YSNs, 13 C NMR spectrum of PS-SO 3 H@ meso silicas DSNs clearly shows the signal at around 142 p.p.m., which could be assigned to the aromatic carbon coordinated with SO 3 H groups, confirming the successful sulphonation ( Supplementary Fig. 2 ). The 29 Si MAS NMR spectrum of PS-SO 3 H@ meso silicas DSNs displays two sets of resonance signals in the range of −35 to −85 p.p.m. and −80 to −120 p.p.m., which are respectively attributed to T and Q silicon species, with a T/(T+Q) of 0.81 calculated by the integration of the peak area. This reveals the coexistence of ethane-silicas and silicas in the outer shell ( Supplementary Fig. 3 ). The above characterizations indicate that PS-SO 3 H@ meso silicas DSNs are hybrid materials composed of PS-SO 3 H, ethane-silicas and silicas. The nitrogen adsorption–desorption isotherms of PS-SO 3 H@ meso silicas DSNs display typical IV isotherm pattern with a sharp capillary condensation step and H4-type hysteresis loop starting from the relative pressure P/P 0 at 0.50 ( Supplementary Fig. 4 ). This indicates the presence of mesopores in the outer shell, according to IUPAC classification (pore diameter of 2.1 nm, similar to YSNs before sulphonation). The existence of the mesopores in the outer shell will benefit the free diffusion of guest molecules throughout the nanospheres. It should be mentioned that the H4 hysteresis in the N 2 sorption isotherm of PS-SO 3 H@ meso silicas DSNs is probably from the hollow interiors of the DSNs [34] , [36] . PS-SO 3 H@ meso silicas DSNs have higher BET surface area (412 m 2 g −1 ) and larger pore volume (0.42 cm 3 g −1 ) than Amberlyst-15 ( Supplementary Table 1 ). Morphology changes with sulphonation time The above results show that the morphology transformation from YSNs to DSNs takes place during the sulphonation process. For clarifying this interesting transformation mechanism, the samples were taken out at desired time intervals during the sulphonation process and characterized by the TEM technique ( Fig. 4 ). At the initial 10 min, only HNs could be observed with similar particle size but thicker shell comparing with PS@ meso silicas YSNs (75 versus 40 nm), and this HNs’ morphology was maintained in the first 2 h. This is probably due to the adherence of dissolved PS to the inner surface of meso silica HNs. Further extending the sulphonation time to 3 h, the inner shell started to appear, and the transformation from HNs to DSNs completed in 4 h. It should be noted that once the inner HNs were completely generated, the outer-shell thickness changed back to 40 nm, similar to that of the initial PS@ meso silicas YSNs. No further changes in morphology could be observed beyond 4 h. The sulphur content increases from 2.1 to 2.4 mmol g −1 as the sulphonation time increases from 1 to 3 h ( Fig. 5a ). After that, the sulphur content tends to be constant, suggesting that the sulphonation reaction nearly completes within 3 h. The acidic exchange capacity of the samples with sulphonation time ≤2 h is nearly identical to the sulphur content, however, it sharply decreases to 1.0 mmol g −1 and levels off after 4 h ( Fig. 5a ). It is worthy to note that the volume of PS-SO 3 H decreased from 8.37 × 10 −21 to 4.61 × 10 −21 m 3 with sulphonation time increasing from 1 to 12 h based on TEM images, showing the aggregation of PS-SO 3 H during the sulphonation process, which cause the percentage of inaccessible sulphonic acid groups to increase from 0.8 to 62.7% ( Fig. 5a ). The above results show that the aggregation of PS-SO 3 H derived by the macromolecular self-assembly within the nanospace of silica HNs during the sulphonation process mainly contributes to the formation of inner HNs. 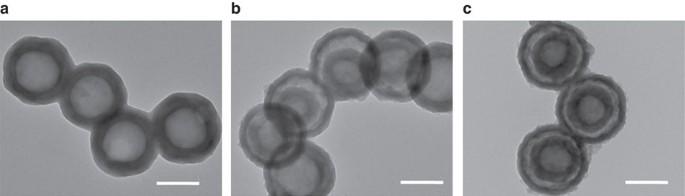Figure 4: Nanostructure evolution with different sulphonation time. (a) TEM images of the samples with sulphonation time of 10 min. Scale bar, 200 nm. (b) TEM images of the samples with sulphonation time of 3 h. Scale bar, 200 nm. (c) TEM images of the samples with sulphonation time of 4 h. Scale bar, 200 nm. Figure 4: Nanostructure evolution with different sulphonation time. ( a ) TEM images of the samples with sulphonation time of 10 min. Scale bar, 200 nm. ( b ) TEM images of the samples with sulphonation time of 3 h. Scale bar, 200 nm. ( c ) TEM images of the samples with sulphonation time of 4 h. Scale bar, 200 nm. 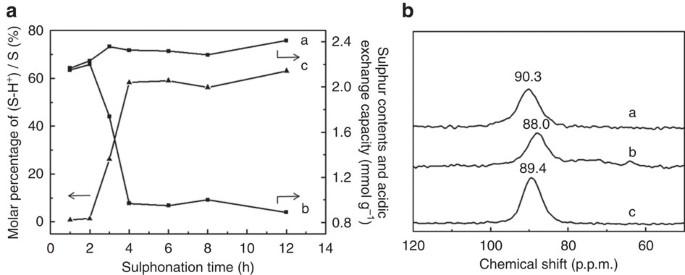Figure 5: Acidity and acid strength characterizations. (a) The sulphur contents (a), acidic exchange capacity (b) and the molar percentage of sulphur to acidic exchange capacity (c) of the samples with different sulphonation time. (b)31P MAS NMR spectra of PS-SO3H@mesosilicas DSNs before (a) and after (b) DMF treatment and Amberlyst-15 (c). Full size image Figure 5: Acidity and acid strength characterizations. ( a ) The sulphur contents (a), acidic exchange capacity (b) and the molar percentage of sulphur to acidic exchange capacity (c) of the samples with different sulphonation time. ( b ) 31 P MAS NMR spectra of PS-SO 3 H@ meso silicas DSNs before (a) and after (b) DMF treatment and Amberlyst-15 (c). Full size image PS-SO 3 H@ meso silicas DSNs are very stable and could maintain the DSN in various nonpolar or polar solvents such as methanol, THF, dioxane, water and pentane ( Supplementary Fig. 5 ). However, in N , N -dimethylformamide (DMF), the morphology of PS-SO 3 H@ meso silicas DSNs changed from DSN to hollow nanostructures ( Supplementary Fig. 6 ). Interestingly, the HNs could be reversibly transformed back to the DSNs by treating with ClSO 3 H. The reversible transformation process could be repeated for several times by alternative DMF and ClSO 3 H treatment ( Supplementary Fig. 6 ). It was found that not only DMF but also pyridine can induce the transformation of HNs to DSNs ( Supplementary Fig. 5 ). In addition to ClSO 3 H, trifluoroacetic acid and p -toluene sulphonic acid could also induce the reversible transformation back to the DSNs ( Supplementary Fig. 6 ). It seems that the above transformations are related with H-bond interactions. H-bond interactions For investigation of H-bond interactions in PS-SO 3 H@ meso silicas DSNs, 1 H MAS NMR technique [37] , [38] , [39] , a useful and direct method for characterizing H-bond interactions in both liquid and solid catalysts, was used. The 1 H MAS NMR spectra of PS-SO 3 H@ meso silicas DSNs and DMF-treated PS-SO 3 H@ meso silicas DSNs display signals at 1.2, 2.7 and 7.4 p.p.m. originated from the protons of -C H -C H - (ethylene group), Si-O H (hydroxyl group) and -Ph H (phenylene group), respectively ( Supplementary Fig. 7 ). The signals at 13.5 p.p.m. should be derived from the protons of SO 3 H groups. However, the proton signal of SO 3 H group cannot be observed in the 1 H NMR spectrum of PS-SO 3 H@ meso silicas DSNs. After DMF treatment, the chemical shift at 13.5 p.p.m. assigned to the proton of sulphonic group [19] was observed. Generally, the higher chemical shift suggests stronger H-bond interactions among adjacent SO 3 H groups. Therefore, the absence of proton signals of SO 3 H for PS-SO 3 H@ meso silicas DSNs may possibly be due to strong H-bond interactions as a result of the aggregation of PS during the sulphonation process. This suggests that strong H-bond interactions exist in PS-SO 3 H@ meso silicas DSNs, and DMF treatment could suppress the H-bond interactions. On the basis of the above results, the formation of DSN during the sulphonation process may involve the dissolution of PS cores and the self-assembly of sulphonated PS driven by H-bond interactions within the confined nanospace of silica HNs. During the sulphonation process, the PS swells and readily dissolves in CH 2 Cl 2 . However, the dissolved species could not escape out of the silica shell. Along with the sulphonation degree of PS increasing, the H-bond interactions among adjacent SO 3 H groups are strengthened and subsequently trigger the self-assembly of PS-SO 3 H within the nanospace of silica HNs. In a control experiment, the sulphonation of PS in CH 2 Cl 2 solution results in no solid products. Thus, the self-assembly of PS-SO 3 H to form aggregated HNs strongly depends on the confined nanospace, which may restrict the free movement of swelled PS-SO 3 H and enhance H-bond interactions owing to the high local concentration of PS-SO 3 H. The treatment of PS-SO 3 H@ meso silicas DSNs in aprotic polar solvents such as DMF and pyridine could destroy H-bond interactions between sulphonic acid groups. The expansion of PS-SO 3 H occurs due to the swelling effect in CH 2 Cl 2 , which causes the formation of HNs. The further treatment of HNs with acids will help to restore the H-bond interactions among sulphonic acid groups. Thus, the aggregation of PS-SO 3 H results in the transformation of HNs back to DSNs. The above results suggest that H-bond interactions play an important role in the morphology transformation of PS-SO 3 H. The TG curves of PS-SO 3 H HNs (obtained by HF treatment of PS-SO 3 H@ meso silicas DSNs), PS-SO 3 H@ meso silicas DSNs and DMF-treated PS-SO 3 H@ meso silicas DSNs exhibit three consecutive weight loss steps in the range of 30–600 °C ( Supplementary Fig. 8 ), which is due to the loss of the physically adsorbed water, decomposition of sulphonic acids and destruction of polymer framework, respectively (the decomposition of ethane-silica in the shell of PS-SO 3 H@ meso silicas DSNs takes place at temperature above 400 °C (ref. 40 )). The decomposition temperature of sulphonic acids of PS-SO 3 H@ meso silicas DSNs is 47 °C higher than that of PS-SO 3 H HNs, probably due to the protective effect of the shell. After treatment with DMF, the decomposition of sulphonic acids starts at lower temperature than that of the fresh PS-SO 3 H@ meso silicas DSNs (264 versus 294 °C). This suggests that H-bond interactions could enhance the thermal stability of sulphonic acids. The previous reports have shown that H-bond interactions could influence the acid strength of solid acids [19] , [41] . Therefore the acid strength of Amberlyst-15, PS-SO 3 H@ meso silicas DSNs as well as DMF-treated PS-SO 3 H@ meso silicas DSNs was investigated using TEPO (triethylphosphine oxide) as a probe molecule in combination with 31 P MAS NMR technique ( Fig. 5b ). The 31 P chemical shift of TEPO chemisorbed on the acid site is sensitive to acid strength, and stronger acid strength will usually lead to larger 31 P chemical shift of TEPO [42] , [43] , [44] . The 31 P NMR spectrum of Amberlyst-15 exhibits a signal at 89.4 p.p.m. that can be assigned to TEPO adsorbed on SO 3 H acid sites. The signal at 90.3 p.p.m. was observed in the 31 P NMR spectrum of PS-SO 3 H@ meso silicas DSNs. The downshift of the signal indicates that PS-SO 3 H@ meso silicas DSNs have stronger Brönsted acid strength than Amberlyst-15. However, the corresponding 31 P NMR signal of DMF-treated PS-SO 3 H@ meso silicas HNs shows an upshift to 88.0 p.p.m., suggesting the decrease in acid strength. In combination with 1 H NMR results, the enhancement and decrease in the acid strength are probably related with H-bond interactions. On the basis of the fact that an increase in the proximity of acid moieties will increase the acid strength due to the site cooperation effect by the formation of H-bond interactions between adjacent acid pairs [22] , it could be deduced that the enhanced acid strength could be attributed to strong H-bond interactions, which can increase the cooperation effect by drawing SO 3 H groups closer. The acid strength of the samples was also measured using ammonia adsorption calorimetry method ( Table 1 and Supplementary Fig. 9 ). The concentration of acid sites measured by ammonia adsorption was similar to that measured using titration method for Amberlyst-15 and Nafion NR50. However, the ammonia adsorption method affords much lower acid sites than titration method for PS-SO 3 H@ meso silicas HNs and DMF-treated PS-SO 3 H@ meso silicas DSNs. The above two samples both have hollow nanostructure. Some of the surface acid sites could form H-bond with the surface hydroxyl group of the organosilica shell and thus could not react with ammonia. The higher acid sites measured by ammonia adsorption method than those by titration method for PS-SO 3 H@ meso silicas DSNs is probably due to the H-bond breakage effect of ammonia, which decreases the aggregation degree of PS-SO 3 H. An average value for ΔH 0 ads (NH 3 ) was calculated and used to measure the acid strength of different samples ( Table 1 ). ΔH 0 ads (NH 3 ) value of PS-SO 3 H@ meso silicas DSNs was about 130 kJ mol −1 , which is lower than Nafion NR50 (ref. 45 ) but higher than Amberlyst-15. In comparison with PS-SO 3 H@ meso silicas HNs, PS-SO 3 H@ meso silicas DSNs afford higher ΔH 0 ads (NH 3 ) value, showing a remarkable enhancement in the acid strength by the formation of double-shell hollow nanostructure. After the DMF treatment, the obvious decrease in ΔH 0 ads (NH 3 ) suggests that the acid strength became weaker probably because of the suppressing of H-bond interactions. The above results suggest that the acid strength of PS-SO 3 H could be tuned by the morphology transformation within the confined nanospace of silica HNs. This provides a new approach to control the acid strength of PS-SO 3 H, which is commonly achieved by varying the chemical compositions and the acid loading. Table 1 The acid strength and acid concentrations*. Full size table The catalytic performance of PS-SO 3 H@ meso silicas DSNs was tested in several important acid-catalysed liquid-phase reactions, such as esterification of fatty acid, Friedel–Crafts alkylation of toluene and CHP (cumene hydroperoxide) cleavage ( Fig. 6 ), and compared with those of Nafion NR50, Amberlyst-15 and H 2 SO 4 ( Table 2 ). The esterification of fatty acids with alcohol to produce esters represents an important pretreatment step in the production of biodiesel from high free fatty acid feedstocks. In the esterification of lauric acid with ethanol, all the acid catalysts show catalytic activity with ethyl laurate as the only product. H 2 SO 4 gives a yield of 71.7% with turnover frequency (TOF) of 31.9 h −1 and Amberlyst-15 affords a yield of 40.2% with TOF of 2.4 h −1 . The low activity of Amberlyst-15 is probably due to the low exposing degree of the active sites to substrates (the BET surface area of Amberlyst-15 is only 45 m 2 g −1 ). Under similar reaction conditions, PS-SO 3 H@ meso silicas DSNs reach a yield of 89.7% with TOF of 28.6 h −1 . The higher yield of ethyl laurate on PS-SO 3 H@ meso silicas DSNs than on H 2 SO 4 (89.7% versus 71.7%) suggests that the unique DSN including hydrophobic -CH 2 -CH 2 - in the outer shell may prevent to some extent the water (formed during the esterification reaction) poisoning the acid sites. PS-SO 3 H@ meso silicas DSNs show much higher activity than PS-SO 3 H HNs, PS-SO 3 H@ meso silicas HNs (obtained with sulphonation time of 3 h) and DMF-treated PS-SO 3 H@ meso silicas DSNs, showing that the external mesoporous organosilica shells and high acid strength [45] benefit for improving the catalytic activity. The organosilica shell may help to stabilize the hollow structure of PS-SO 3 H during the catalytic process. It should be mentioned that the sulphonated silica HNs exhibit only 4.9% conversion of lauric acid, showing that almost no sulphonic acid group could be incorporated in the shell during the sulphonation process. 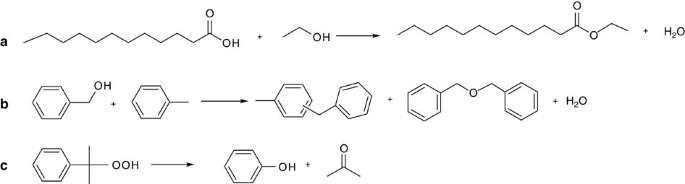Figure 6: Acid-catalysed liquid-phase reactions. (a) Esterification of fatty acid. (b) Friedel–Crafts alkylation of toluene. (c) Cumene hydroperoxide cleavage. Figure 6: Acid-catalysed liquid-phase reactions. ( a ) Esterification of fatty acid. ( b ) Friedel–Crafts alkylation of toluene. ( c ) Cumene hydroperoxide cleavage. Full size image Table 2 Catalytic activity and selectivity. Full size table The catalytic performance of different samples was also tested in Friedel–Crafts alkylation of toluene by benzyl alcohol, an important industry process to produce diphenyl compounds that are essential intermediates for pharmaceutical and fine chemical production [46] , [47] , [48] . All acid catalysts could catalyse this reaction with methyl diphenylmethanes as desired product and dibenzyl ether as side product ( Supplementary Fig. 10 ). At an S/C of 57.5, H 2 SO 4 shows a very low activity (4.9% conversion with 50.1% selectivity to methyl diphenylmethanes). Only at high catalyst concentration (an S/C of 5), H 2 SO 4 could afford 96.2% conversion with 78.8% selectivity to methyl diphenylmethanes. This suggests that high concentration of liquid acid is necessary for achieving desired activity. At an S/C of 57.5, PS-SO 3 H@ meso silicas DSNs that give 99.1% conversion with 72.8% selectivity to methyl diphenylmethanes are much more active and selective than H 2 SO 4 and Amberlyst-15. The fact that PS-SO 3 H@ meso silicas DSNs are less selective than Nafion NR50 but more selective than PS-SO 3 H@ meso silicas HNs and DMF-treated PS-SO 3 H@ meso silicas DSNs suggests that higher acid strength could result in higher selectivity. The low activity and selectivity of PS-SO 3 H HNs once again confirm the importance of the organosilica shell for obtaining high activity and selectivity. In acid-catalysed cleavage of CHP into phenol and acetone, PS-SO 3 H@ meso silicas DSNs afford 99.5% conversion with 99.8% selectivity to phenol, which was much higher than PS-SO 3 H HNs, DMF-treated PS-SO 3 H@ meso silicas DSNs and Amberlyst-15. Considering dangerous explosive problem, the catalytic behaviour of H 2 SO 4 was not tested. The above results suggest that the high activity and selectivity of PS-SO 3 H@ meso silicas DSNs are probably attributed to their strong acid strength, high local concentration of active sites and unique DSN. The recycle stability of PS-SO 3 H@ meso silicas DSNs was investigated using esterification of lauric acid with ethanol as the model reaction ( Supplementary Fig. 11 ). The solid catalyst could be easily recovered by centrifugation. After being washed and dried, the recovered catalyst was directly used for the next reaction cycle. The fresh solid catalyst gave 93.3% yield of ethyl laurate within 6 h. In the second run, the yield slightly dropped to 87.9% under the same reaction condition. After the second cycle the yield becomes quite steady in the following cycles (for example, 86.6% yield for the eighth cycle), suggesting that PS-SO 3 H@ meso silicas DSNs are stable and could be recycled. After the first cycle, PS-SO 3 H@ meso silicas DSNs have similar morphology as the fresh ones in acid-catalysed reactions, including esterification of fatty acid, Friedel–Crafts alkylation of toluene and CHP (cumene hydroperoxide) cleavage reactions ( Supplementary Fig. 12 ). However, the morphology changes from double-shell HNs to HNs, and the BET surface area and pore volume decrease obviously after eighth cycle in the esterification reaction, probably due to the polymer swelling caused by the reactants and products during the catalytic process and the mesopore blockage by the swelled polymer. In summary, a novel hybrid solid acid with DSN was fabricated on the basis of the self-assembly of PS-SO 3 H resin driven by H-bond interactions among SO 3 H groups within the nanospace of silica HNs. Interestingly, it was found that the acid strength of PS-SO 3 H@ meso silicas DSNs could be enhanced and decreased by restoring and destroying H-bond interactions, respectively. PS-SO 3 H@ meso silicas DSNs with enhanced acid strength and unique double-shell mesostructure show excellent catalytic activity and selectivity in a series of important acid-catalysed reactions. Our findings may offer a new approach to fabricate highly efficient solid acid catalysts for green chemical processes. Chemicals and reagents All materials were of analytical grade. Styrene was washed through an inhibitor remover column for removing the inhibitor and then distilled under vacuum before use. The other materials were used as received without any further purification. 1,2-Bis-(trimethoxysilyl)ethane (BTME), cetyltrimethylammonium bromide (CTAB) and triethylphosphine oxide (TEPO) were purchased from Sigma-Aldrich Company Ltd. (USA). Fluorocarbon surfactant, FC-4, was bought from YickVic Chemicals (Hong Kong). Tetraethoxysilane (TEOS) was obtained from Nanjing Shuguang Chemical Group (China). Other reagents were purchased from Shanghai Chemical Reagent, Inc. of the Chinese Medicine Group. Synthesis of polystyrene template spheres The PS template spheres were prepared by emulsion polymerization in a water system according to a modified method [49] . Specifically, PVP (0.55g) was dissolved into 50 ml of deionized water and 6.5 ml of styrene in a flask under vigorous stirring. Then, 0.15 g of K 2 S 2 O 8 dissolved in 20 ml of water was added. Nitrogen was bubbled into the system for 1 h to remove the oxygen from the reactor. Then, reaction mixtures were sustained at 70 °C for 24 h under argon atmosphere. After polymerization reaction, the solution was centrifuged and washed with water and ethanol for three times. The obtained white solid was dried under vacuum at 60 °C overnight. For characterization procedures, see Supplementary Methods . Synthesis of PS@ meso silicas YSNs In the first step, the silica layer was coated on the PS template using the following procedure: a mixture of H 2 O (60 ml), ethanol (20 ml), CTAB (0.2 g), PS template spheres (0.2 g) and NH 3 ·H 2 O (0.7 ml, 25 wt %) was stirred at 50 °C for 0.5 h. Then, TEOS (0.5 g) was added and the mixture was stirred for 2 h, followed by the addition of an aqueous solution (3 ml) containing FC-4 (0.04 g), CTAB (0.08 g) and NH 3 .H 2 O (0.20 ml, 25 wt %). The mixture was stirred for 0.5 h. The second step involves selective etching according to the following procedure: BTME (0.50 ml) in ethanol solution (2 ml) was added subsequently under vigorous stirring to the above synthesis medium. After stirring for 2 min, the temperature was raised to 80 °C and kept for 2 h, and the white powder was collected by filtration and dried at room temperature. To remove the surfactant, the as-synthesized materials (1 g) were dispersed in 200 ml of ethanol containing 1.5 g of concentrated HCl aqueous solution and the mixture was stirred at 70 °C for 12 h. After centrifugation and washing with ethanol, the desired material was obtained. At last, the obtained solid was dried at 60 °C overnight. The resulting powder products were denoted as PS@ meso silicas YSNs. Synthesis of PS-SO 3 H@ meso silicas DSNs Solid acids with DSN were obtained in one-pot step. In a typical procedure, PS@ meso silicas YSNs (1.0 g) were degassed at 120 °C under vacuum for 3 h. Then anhydrous dichloromethane (50 ml)-containing chlorosulphonic acid (10 ml) was slowly introduced at 0 °C. The mixture was stirred at 0 °C for 12 h under argon atmosphere. The suspension was washed with copious amount of water until the filtrate was neutral. After centrifugation and washing with ethanol, the desired material was obtained. Finally, the solid was dried at 60 °C overnight. The resulting powder products were denoted as PS-SO 3 H@ meso silicas DSNs. Treatment of PS@ meso silicas DSNs in different organic solvents To investigate the stability of PS@ meso silicas DSNs, PS@ meso silicas DSNs (0.1 g) were treated in different types of organic solvents (10 ml; the organic solvent includes methanol, THF, ethanol, dioxane, water, pyridine, pentane and DMF) for 12 h under stirring at room temperature. After centrifugation and washing with ethanol, the powder products were dried at 60 °C overnight. General procedure for acid-catalysed reactions Esterification of lauric acid with ethanol was carried out in a two-necked round flask equipped with a reflux condenser and a magnetic stirrer. The catalyst was pretreated at 120 °C under vacuum for 3 h. In a typical experiment, 10 mmol of ethanol and 2 mmol of lauric acid were added to the flask containing 0.05 g of PS@ meso silicas DSNs (0.04 mmol of acid sites). The mixture was stirred at 80 °C for 6 h. The reaction products were collected by a syringe at regular intervals and analysed using a precalibrated gas chromatograph (Agilent 7890) equipped with a flame ion detector (FID) and PEG capillary column (30 m × 0.25 mm × 0.25 μm). Tetradecane was used as an internal standard. Liquid-phase Friedel–Crafts alkylation of toluene by benzyl alcohol was carried out in a two-necked round-bottom flask coupled with a reflux condenser in a temperature-controlled oil bath. In a typical experiment, 0.05 g of PS@ meso silicas DSNs (0.04 mmol of acid sites) catalyst was added to a reactant mixture of 0.25 g of benzyl alcohol in 10.0 ml of toluene, with 0.05 g of tetradecane as an internal standard for the GC analysis. The reaction was refluxed under vigorous magnetic stirring at 80 °C for 7 h. The reaction mixture was monitored using gas chromatography (GC, Agilent-7890A) equipped with a FID and a HP-5 column (30 m × 0.32 mm × 0.25 μm). GC-mass spectrometer (GC–MS) was also used to identify the reaction products. The CHP cleavage reaction was carried out in a round-bottom flask coupled with a reflux condenser in a temperature-controlled water bath. In a typical experiment, 0.01 g of PS@ meso silicas DSNs (8.7 × 10 −3 mmol of acid sites) catalyst was added to 1.0 g of CHP with 0.1 g of tetradecane as an internal standard for GC analysis. The reaction mixture was refluxed under vigorous magnetic stirring at 50 °C for 1 h. The concentration of CHP and phenol was monitored using gas chromatography (GC, Agilent-7890A) equipped with a FID and a HP-5 column (30 m × 0.32 mm × 0.25 μm). The reusability of PS-SO 3 H@ meso silicas DSNs was tested using esterification of lauric acid with ethanol as the model reaction. In a typical experiment, 10 mmol of ethanol and 2 mmol of lauric acid were added to the flask containing 0.10 g of catalyst. The mixture was stirred at 80 °C for 6 h. After the completion of one cycle, the catalyst was filtered from the reaction system, thoroughly washed with ethanol, dried under vacuum at 60 °C overnight and then used in the next cycle. How to cite this article: Zhang, X. et al. Polystyrene sulphonic acid resins with enhanced acid strength via macromolecular self-assembly within confined nanospace. Nat. Commun. 5:3170 doi: 10.1038/ncomms4170 (2014).